Mixtures of planetary ices at extreme conditions The interiors of Neptune and Uranus are believed to be primarily composed of a fluid mixture of methane and water. The mixture is subjected to pressures up to several hundred gigapascal, causing the ionization of water. Laboratory and simulation studies so far have focused on the properties of the individual components. Here we show, using first-principle molecular dynamic simulations, that the properties of the mixed fluid are qualitatively different with respect to those of its components at the same conditions. We observe a pressure-induced softening of the methane–water intermolecular repulsion that points to an enhancement of mixing under extreme conditions. Ionized water causes the progressive ionization of methane and the mixture becomes electronically conductive at milder conditions than pure water, indicating that the planetary magnetic field of Uranus and Neptune may originate at shallower depths than currently assumed. A methane–water fluid mixture may make up more than 90% of the 'icy' middle layers of Neptune and Uranus [1] . The mixture undergoes progressive dissociation and ionization as a function of increasing pressure and temperature (P–T) along the planetary radius, starting from a few tens of gigapascals and a few thousand degrees kelvin [2] . The ionic fluid is believed to be responsible for the magnetic field, about half of the terrestrial value [3] , measured at the planetary surfaces. The relevance of water–methane mixtures in planetary science may extend beyond the solar system, as new extrasolar planets with ice-like compositions are being discovered [4] . Methane-rich hydrous fluids are also ubiquitous in the Earth. Knowledge of their properties is crucial, for example, in the understanding of the abiogenic formation of methane [5] , [6] . H 2 O–CH 4 fluid mixtures exist in the Earth only down to upper mantle conditions, that is, at milder P–T conditions than in giant planets; however, knowledge of their properties throughout a much wider range can help constrain thermodynamic models at the relevant geothermal conditions. At low temperature and high pressure, methane–water mixtures crystallize into stable clathrate structures [8] , [9] , wherein methane guest molecules occupy the cages of a host network of hydrogen-bonded water molecules. From a fundamental perspective, extreme conditions can be seen as an efficient way to probe the repulsive region of the intermolecular potential at unconventionally short distances. Diffraction experiments on methane clathrate hydrates, for example, show a considerable shortening of the C–O distances already at 3 GPa (ref. 8 ) to values compatible with the existence of hydrogen bonding between CH 4 —a nominally apolar molecule—and H 2 O, suggesting qualitative pressure-induced changes in the chemical interaction between the two species with respect to ambient conditions. At higher pressures, reduction of the intermolecular distances leads, in pure water, to hydrogen-bond symmetrization in ice and to ionization in the fluid [10] . Ionization turns hot dense water into a highly corrosive solvent [11] with remarkable catalytic properties [12] . From a planetary science perspective, laboratory and simulation studies have now focused on the properties of the individual components, water [2] , [10] , [13] , [14] , [15] , [16] , [17] , [18] and methane [19] , [20] , [21] , [22] , [23] . But pressure- and temperature-induced chemical interactions may qualitatively change the properties of the mixtures with respect to those of the individual components. For example, diamond formation in icy planets is inferred from studies based on hydrocarbon dissociation in the absence of water [19] , [20] , [21] , [23] . Similarly, estimates of the electrical conductivity in the planetary cores are essentially based on studies on pure water [2] , [13] , [14] , [15] , [16] , [17] , with the only exception of a study carried out on the mixture up to 77 GPa (ref. 13 ), which is at the lower end of the region of pressure where water is dissociated. These studies yield conductivities typical of an ionic fluid throughout most of the planetary radius, with evidence for metallic behaviour only in the deepest regions of the planets, close to the core. However, recent planetary models would be more compatible with metallic-like conductivities in the icy layer [24] , suggesting qualitative differences in the electrical properties of the mixture, with respect to pure water. From a theoretical standpoint, water–methane mixtures have been studied up to 2,500 K and 18 GPa by atomistic simulations based on empirical force fields [7] . Such force fields assume intact molecules and cannot be extended to more extreme conditions in which chemical dissociation takes place. On the other hand, first-principle simulations based on density-functional theory have successfully described the self-ionization of pure water [14] , [15] , [16] and the catalytic activity of dense hot water in detonation processes [12] . In this paper we study the properties of CH 4 /H 2 O mixtures at extreme conditions by means of density-functional theory-based first-principle molecular dynamics (MD). We consider four P–T conditions: 15 GPa and 1,800 K, 50 GPa and 3,000 K, 120 GPa and 4,000 K, and 300 GPa and 5,000 K. The first two P–T points are representative of an undissociated and a partially dissociated regime for water, respectively. The last two P–T points correspond to fully dissociated water. According to conductivity measurements on pure H 2 O (ref. 17 ), the second and third conditions correspond to a semiconducting behaviour, whereas the fourth condition corresponds to an electronic conductor. 15 GPa and 1,800 K At 15 GPa and 1,800 K, water is on the verge of dissociation, with a few dissociation events observed consisting in the formation of transient H 3 O + –OH − complexes. This behaviour is similar to the one observed in pure water [15] . Methane instead appears to be chemically stable. From a pair-correlation analysis ( Fig. 1 ), we find that the average C–O distance at these conditions is 2.9 Å. Such a distance is in principle compatible with hydrogen-bond formation between water and methane. A visual examination of selected snapshots along the simulation shows that, in their approaches to water, methane molecules distort considerably and form H 3 CH...OH 2 and H 4 C...HOH motifs in roughly equal proportions. However, at 1,800 K, molecular distortion is so pronounced that a pure geometrical analysis of the nature of the bond becomes difficult. To quantify the effects of molecular distortion we calculated the time-dependent dipole moment acquired by methane molecules along the trajectory, using the Wannier-function method [25] . Although the methane dipole moment averages to zero with time, as expected for an apolar system, the distortion from ideal tetrahedral coordination causes methane to acquire an instantaneous dipole moment with an average absolute value of 0.5 Debye at these conditions ( Fig. 2a ). Moreover, the positions of the Wannier-function centres along the C–H bonds are slightly displaced towards carbon, with respect to their positions calculated for the isolated molecule as shown in Figure 2b . 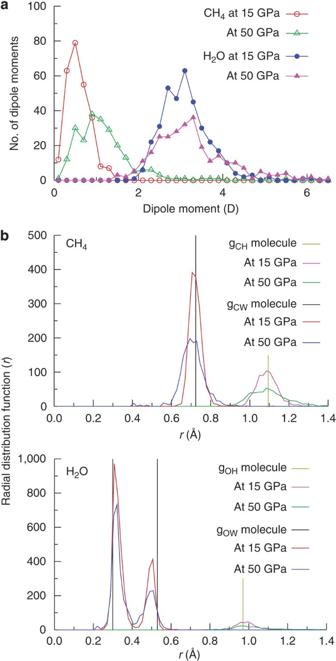Figure 2: Methane acquires a dipole moment under pressure. (a) Histogram of the absolute value of the molecular dipole moments of CH4and H2O at 15 GPa and 1,800 K and at 50 GPa and 3,000 K. (b) Radial distribution functions (RDFs) between Wannier function centres and carbon (upper panel) and oxygen (lower panel). Also shown are the RDFs between carbon (oxygen) and the corresponding protons in methane (water). For reference, results for the isolated molecules are reported as vertical lines. This indicates that the polarity of the individual C–H bonds is also slightly increased with respect to the gas-phase value. We conclude that the combined effect of P–T causes methane to depart significantly from the symmetric, apolar picture typical of its behaviour at ambient conditions. The molecular distortion and the consequent formation of an instantaneous dipole moment soften the repulsive region of the water–methane intermolecular potential and explain the short C–O distances observed in our simulations. On the other hand, the presence of methane does not seem to qualitatively affect the hydrogen-bonding properties of water. The strength of the hydrogen bonding in pure water can be monitored by analysing changes in the strength of the second peak (first intermolecular peak) of the O–H pair distribution function [15] . A comparison between the O–H pair correlation function in the mixture at 15 GPa and 1,800 K ( Fig. 1 ) and that of pure water at 14.5 GPa and 750 K (ref. 15 ) points to a reduction in the strength of the second peak upon mixing with methane. The reduction is, however, consistent with the higher temperature of the simulation for the mixture and with the reduction in the number of water molecules in the first coordination shell, because of the presence of methane. 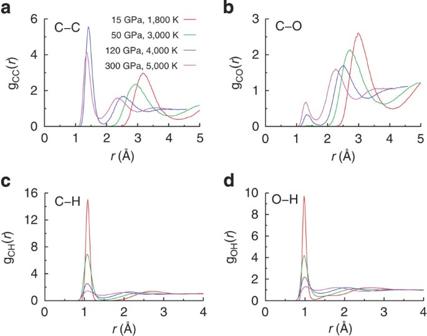We conclude that the strength of the water–water hydrogen bond in pure water and in the mixture is qualitatively similar. Figure 1: Radial distribution functions. Radial distribution functions g(r) as a function of the distance between atom pairs: (a) C–C, (b) C–O, (c) C–H and (d) O–H. Colour codes represent different pressure–temperature conditions and are the same for the four panels. Figure 1: Radial distribution functions. Radial distribution functions g( r ) as a function of the distance between atom pairs: ( a ) C–C, ( b ) C–O, ( c ) C–H and ( d ) O–H. Colour codes represent different pressure–temperature conditions and are the same for the four panels. Full size image Figure 2: Methane acquires a dipole moment under pressure. ( a ) Histogram of the absolute value of the molecular dipole moments of CH 4 and H 2 O at 15 GPa and 1,800 K and at 50 GPa and 3,000 K. ( b ) Radial distribution functions (RDFs) between Wannier function centres and carbon (upper panel) and oxygen (lower panel). Also shown are the RDFs between carbon (oxygen) and the corresponding protons in methane (water). For reference, results for the isolated molecules are reported as vertical lines. Full size image 50 GPa and 3,000 K At 50 GPa and 3,000 K, methane starts dissociating under the effect of an almost completely ionized water. The C–H pair correlation function ( Fig. 1 ) is still characterized by a well defined peak, but the lifetime of the C–H bond, estimated on the basis of a cutoff radius of 1.5 Å, is found to be about 50 fs, about four times the C–H-bond stretching period. Water dissociation is instead almost complete. Proton jumps occur between both carbon and oxygen with an overall diffusion constant for the proton of 1.3×10 −3 cm 2 s −1 , comparable to that observed in pure water [14] . The formation of a few C–O bonds is observed during the simulation, with a lifetime of more than 0.5 ps, one of them lasting through the last 3 ps of the simulation. Formation of C–C bonds is not observed at these conditions. In the case of pure CH 4 , methane dissociation is accompanied by the formation of mixtures of more complex saturated hydrocarbons [6] , [21] , [26] . Our results for the mixture suggest that the presence of water prevents the formation of complex carbon species, at least at 50 GPa and 3,000 K. Except for a few C–O bonds, none of the other chemical bonds appear to be stable throughout a large portion of the simulation. 120 GPa and 4,000 K At 120 GPa and 4,000 K, we observe the full dissociation of methane and the formation of several C–C and C–O bonds ( Fig. 1 ). C–C bonds have a lifetime of 3.5 ps and form small transient complexes consisting of 2–4 carbon atoms. The transient formation of H 2 molecules is also observed. The conductivity of pure water at similar conditions is known to be far from metallic at these conditions [16] , [17] . However, the density of electronic states extracted from our simulations indicates an almost vanishing excitation energy already at 50 GPa, and full gap closure at 120 GPa ( Fig. 3 ), a behaviour consistent with metallicity at milder conditions than in pure water. The remarkable difference between pure water and the mixture can be traced to the ionic nature of the water fluid, compared with the covalent nature of the C–H bonds. Bond breaking and reforming lead to a proliferation of states crossing the Fermi level. Such transient electronic states may be localized and therefore not leading, in strict terms, to a fully metallic behaviour, but their presence will enhance the electronic contribution to the conductivity and may dominate over the ionic contribution. 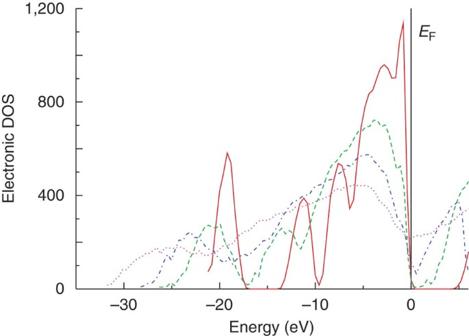Figure 3: Metallic behaviour at extreme conditions. Electronic density of states (DOS) of the mixture at different pressure–temperature conditions.EFindicates the Fermi energy. The red solid line corresponds to 15 GPa and 1,800 K, the green dashed line corresponds to 50 GPa and 3,000 K, the blue dot-dashed line corresponds to 120 GPa and 4,000 K and the pink dotted line corresponds to 300 GPa and 5,000 K. Figure 3: Metallic behaviour at extreme conditions. Electronic density of states (DOS) of the mixture at different pressure–temperature conditions. E F indicates the Fermi energy. The red solid line corresponds to 15 GPa and 1,800 K, the green dashed line corresponds to 50 GPa and 3,000 K, the blue dot-dashed line corresponds to 120 GPa and 4,000 K and the pink dotted line corresponds to 300 GPa and 5,000 K. Full size image 300 GPa and 5,000 K At 300 GPa and 5,000 K, dissociation is complete. Several C–C bonds are formed, together with occasional C–O bonds. C–C bonds form and break in a dynamic manner, leading to transient carbon complexes with carbon atoms in different coordinations, up to fourfold, that is, diamond-like, but with an average C–C coordination of only 1.4 (to be compared with 1.2 at 120 GPa). The average coordination is reached in the first few picoseconds of the simulation, and remains constant throughout the next 15 ps, despite several bond-breaking and -forming events. The short duration of our simulation does not allow us to rule out the possibility that on longer time scales carbon could segregate and form diamond. However, in simulations of pure methane at similar conditions [20] , the formation of C–C bonds was an irreversible process and none of the newly formed C–C bonds was observed to break after being formed. In the present study of methane in water, none of the chemical bonds persists for the full duration of the simulation. Diamond precipitation is therefore not incompatible with the present results, but it is challenged by the microscopic evidence that, contrary to pure methane, chemical bonds are unstable in the mixture. At 300 GPa and 5,000 K, the electronic density of states is characteristic of a standard metal, with a density of states at the Fermi level roughly half that of its maximum. This is qualitatively different with respect to early simulations on pure water, where the density of states at the Fermi level was much smaller at the same conditions [14] . Our simulations suggest that mixing leads to remarkable changes in the response of methane and water to extreme conditions, with respect to the behaviour of the pure substances. Before dissociation, methane acquires a significant fluctuating dipole moment that causes a reduction of the methane–water repulsion. It is generally assumed that a shortening of the characteristic length between unlike species (in comparison with like species) favours mixing in a binary fluid. This is, for example, the case of hard spheres, arguably the simplest interparticle potential [27] . 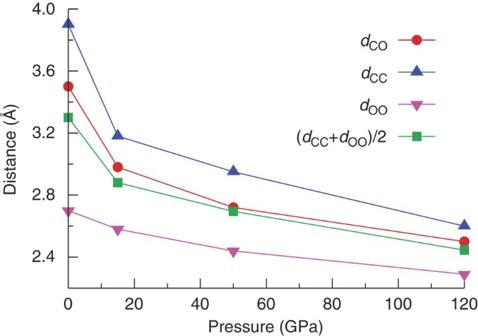Figure 4: Intermolecular distances. Average distances between oxygen atoms for water (triangle down), between carbon atoms for methane (triangle) and between carbon and oxygen (circle). Data at ambient pressure are taken from ref.28for water–water, from ref.29for water–methane and from ref.30for methane–methane in water. Data at high pressures are calculated from the intermolecular peak of the radial distribution functions shown inFigure 1. Also shown is the water–methane distance expected for an ideal additive mixture (square). As shown in Figure 4 , water–methane intermolecular distances fall more rapidly than expected on the basis of the ideal additivity rule. The higher melting temperature observed at high pressure for methane clathrates with respect to pure water and methane [31] and the stability of methane clathrates to almost megabar pressures [9] are both consistent with the softening of the repulsive component of the methane–water intermolecular potential, which points to an increased propensity of methane to form mixed phases with water under compression. C–O distances compatible with hydrogen bonding were also observed in methane hydrate clathrates [8] compressed to 3 GPa at room temperature. Pressure-induced distortion of the methane molecules may also explain the short distances observed in the solid phases. Intermolecular models used so far to determine the equations of state of methane–water fluid mixtures are based on rigid molecules [7] and may be unable to describe mixing above a few GPa. At more extreme conditions, we find that the mixture becomes electronically conducting at pressures below 120 GPa, where pure water is reported to be still an opaque semiconductor [17] . Because electronic conductivity generally dominates over the ionic contribution, the source of the planetary magnetic fields observed at Uranus and Neptune may be shallower than currently inferred from conductivity data on pure substances, in agreement with revised planetary models [24] . Our simulations also indicate that ionized water is, not surprisingly, an exceptionally aggressive chemical solvent, capable of dissociating methane already at 50 GPa. However, contrary to pure methane, CH 4 dissociation is followed by the formation of more complex carbon compounds only at the highest pressures in this study. At 50 GPa, ionized methane is still fully soluble, yet in a partially ionized form, in fully ionized water. Our findings call for a revision of composition models for the interiors of icy giant planets, in particular those based on the behaviour of pure hydrocarbons and implying diamond formation. They also underscore the importance of the chemical environment in the pressure-induced dissociation of methane, as already noted in the study by Kolesnikov et al [6] . In the near future, shockless compression experiments [32] are expected to reach the conditions of P–T described in this work. Reflectivity and equation-of-state measurements could test the validity of our predictions. Figure 4: Intermolecular distances. Average distances between oxygen atoms for water (triangle down), between carbon atoms for methane (triangle) and between carbon and oxygen (circle). Data at ambient pressure are taken from ref. 28 for water–water, from ref. 29 for water–methane and from ref. 30 for methane–methane in water. Data at high pressures are calculated from the intermolecular peak of the radial distribution functions shown in Figure 1 . Also shown is the water–methane distance expected for an ideal additive mixture (square). Full size image Computational details The mixture was simulated by means of density-functional-theory-based MD in the Car-Parrinello approximation [33] , using the Quantum-Espresso package [34] . The simulated mixture composition (26 CH 4 /38 H 2 O molecules) is representative of a typical planetary composition. The starting configuration at each condition was generated by means of classical MD simulations [35] . The Perdew-Burke-Ernzerhoff exchange-correlation functional [36] and norm-conserving pseudopotentials were used together with a plane wave basis set for the electronic wave functions. An energy cutoff of 80 Ry was used for the plane wave basis set. The stress tensor was corrected for basis set non-completeness by repeating its calculation with a cutoff of 240 Ry at selected points along the trajectory. Temperature was kept constant by means of a Nose-Hoover thermostat. The mixture was equilibrated for about 2 ps and then simulated for at least 20 ps at each P–T point. The electronic fictitious masses for the Car-Parrinello dynamics and the time steps are fixed at 200 a.u. and 0.0726 fs for 15 GPa/1,800 K, at 160 a.u. and 0.0484 fs for 50 GPa/3,000 K, at 120 a.u. and 0.0363 fs for 120 GPa/4,000 K and at 100 a.u. and 0.0242 fs for 300 GPa/5,000 K after careful examination for each P–T condition. Analysis The vibrational density of states was determined from the Fourier transform of the velocity–velocity time correlation function. The instantaneous molecular dipole was obtained as , where N is the number of atoms in a molecule, q i is t he valence atomic charge of atom i and R WS are the four Wannier centre positions associated with each molecule [25] . How to cite this article: Lee, M.-S. & Scandolo, S. Mixtures of planetary ices at extreme conditions. Nat. Commun. 1:185 doi: 10.1038/ncomms1184 (2011).